Histone H3.3 and its proteolytically processed form drive a cellular senescence programme The process of cellular senescence generates a repressive chromatin environment, however, the role of histone variants and histone proteolytic cleavage in senescence remains unclear. Here, using models of oncogene-induced and replicative senescence, we report novel histone H3 tail cleavage events mediated by the protease Cathepsin L. We find that cleaved forms of H3 are nucleosomal and the histone variant H3.3 is the preferred cleaved form of H3. Ectopic expression of H3.3 and its cleavage product (H3.3cs1), which lacks the first 21 amino acids of the H3 tail, is sufficient to induce senescence. Further, H3.3cs1 chromatin incorporation is mediated by the HUCA histone chaperone complex. Genome-wide transcriptional profiling revealed that H3.3cs1 facilitates transcriptional silencing of cell cycle regulators including RB/E2F target genes, likely via the permanent removal of H3K4me3. Collectively, our study identifies histone H3.3 and its proteolytically processed forms as key regulators of cellular senescence. Cellular senescence is a stable form of growth arrest and is thought to function as a potent anti-tumour mechanism [1] , [2] . Cellular senescence was originally defined as ‘replicative exhaustion’ that occurs in cultured cells over time, but can also be provoked prematurely by stresses that include DNA damage and activated oncogenes [3] , [4] , [5] . For example, melanocytes within human nevi often harbour an activating mutation in BRAF (BRAF V600E ) and can remain senescent for decades [6] . Characteristic features of senescent cells include morphological and physiological alterations, senescence-associated β-galactosidase (SA-β-gal) activity, chromatin condensation and extensive gene expression changes [4] , [7] . Senescence is mediated by the RB and p53 pathways, which cooperate to ensure cell cycle inhibition [7] , [8] , [9] . A growing body of evidence suggests that the process of cellular senescence is also mediated by chromatin changes [10] , [11] , [12] , [13] , [14] , [15] . Notably, senescent human cells often accumulate distinct 4′,6-diamidino-2-phenylindole (DAPI)-dense nuclear foci known as senescent-associated heterochromatin foci (SAHF). SAHF are enriched for repressive chromatin modifications such as H3K9me3 and H3K27me3, chromatin architectural factors such as high mobility group A (HMGA) proteins, and the histone variant macroH2A [11] , [12] , [13] . Interestingly, SAHF formation is not driven by a redistribution of histone post-translational modifications (PTMs) in the senescent genome, but rather a spatial reorganization of existing repressive PTMs [14] . The deposition of macroH2A is a late step in SAHF formation and is dependent on components of the H3.3 histone chaperone complex HUCA (HIRA/UBN1/CABIN1/ASF1a) [12] . Interestingly, ectopic expression of HIRA or ASF1a alone or together can induce senescence; however, the role of H3.3 in driving a senescence programme remains unclear. Recently, we mapped the histone PTM profile of senescent cells [15] . We identified a striking loss of H3K4me3, a PTM associated with active transcription, at E2F target genes. We further identified the H3K4 demethylases JARID1A and JARID1B to be responsible for the removal of H3K4me3. In addition to the action of histone-modifying enzymes, the incorporation of histone variants and the proteolytic processing of histones have also emerged as mechanisms that alter the histone PTM landscape [16] . In fact, proteolytic processing of histone H3 has been reported in the heterochromatic micronuclei of Tetrahymena [17] and during embryonic stem cell (ESC) differentiation via the lysosomal protease Cathepsin L1 (CSTL1) [18] . However, a clear biological function for such histone tail processing has yet to be elucidated. In this study, we report evidence of H3 tail proteolytic processing in models of both oncogene-induced and replicative senescence. We identified two distinct processing sites of the H3 tail, both of which are mediated by CTSL1. One of these sites, H3cs1, corresponds to the cleavage site identified in differentiating ESCs, which generates a new H3 tail beginning at amino-acid T22 (ref. 18 ). We find a chromatin-bound pool of the active CTSL1 protease, which correlates with the emergence of cleaved H3 products during senescence. We demonstrate that the histone variant H3.3 is cleaved during senescence and that ectopic expression of H3.3, and to a greater extent H3.3cs1, induces senescence in the absence of oncogenic signalling. Further, the chromatin incorporation of endogenous cleaved H3 during oncogene-induced senescence (OIS) and ectopic H3.3cs1 requires the HUCA complex. RNA-sequencing (RNA-seq) studies revealed that introduction of H3.3cs1 into primary fibroblasts results in rapid transcriptional downregulation of cell cycle genes, with significant overlap of those downregulated during OIS. H3.3cs1-downregulated genes also significantly overlap with genes that lose H3K4me3 during senescence, many of which are RB and JARID1A/1B targets [15] . Together, these findings suggest that H3 tail cleavage functions as a key mechanism to remove H3K4me3, and thereby contributes to the silencing of cell cycle-promoting genes during senescence. Senescent fibroblasts show nucleosomal forms of cleaved H3 RAS-induced senescence (ER::H-RAS G12V ) in IMR90 fibroblasts is a well-characterized system in which senescence is enforced by the combined action of the RB and p53 tumour-suppressor pathways [9] , [19] . Using this system, we induced senescence by the addition of 4-hydroxytamoxifen (4OHT) to primary fibroblasts and assayed cells for established senescence markers ( Fig. 1a ; Supplementary Fig. 1 ). Consistent with our previous findings [15] , we detected a striking loss of H3K4me3 during senescence ( Fig. 1b ). Upon immunoblotting for histone PTMs such as H3K14 and H3K18 acetylation, we noted not only an expected decrease of these marks, but also a faster running species of H3 ( Fig. 1b , asterisks). Immunoblotting of PTMs more distal in the tail (H3K27me3 or H3K36me3) or with a C-terminal H3 antibody, revealed an additional faster-migrating species of H3 ( Fig. 1b , arrows). These faster-migrating species appeared with increasing intensity over a senescence time course of ~2 weeks, but were not detected with antibodies specific for PTMs at the N terminus of the H3 tail, such as H3K4me3 and H3K9me3. No evidence of H4 cleavage was detected either ( Fig. 1b ). Collectively, these results suggested that the N-terminal tail of H3 is specifically cleaved during OIS at two distinct sites. 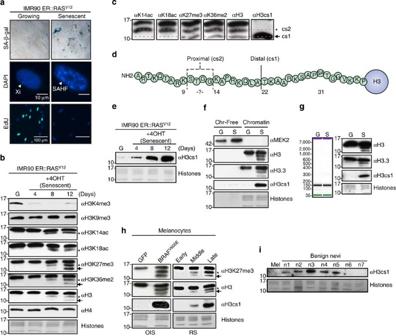Figure 1: Histone H3 tail is processed upon oncogene-induced senescence in fibroblasts and melanocytes. (a) Inducible RASV12-driven OIS system in IMR90 fibroblasts evidenced by SA-β-Gal staining ( × 10 images shown), DAPI staining to monitor SAHF formation and EdU incorporation. Scale bars as shown. (b) Immunoblots of growing (G) and senescent (S) IMR90s with the indicated histone H3 PTM-specific antibodies. Asterisks indicate the proximal cleavage (cs2) and arrows indicate the distal cleavage (cs1). In all panels, core histones were stained with Amido Black for loading. (c) Immunoblot of the chromatin fraction of senescent IMR90s showing alignment of full-length and cleaved histone H3 products. H3cs1-specific antibody used for alignment of the distal cleavage product. (d) Diagram of histone H3 tail showing cleavage sites. Dashed lines indicate potential proximal cleavage (cs2) sites, as determined by immunoblotting with H3 PTM-specific antibodies. The solid line marks the distal cleavage site (cs1). (e) Immunoblot of growing and senescent IMR90 cells with a cleavage-specific antibody (αH3cs1), which recognizes the N terminus of H3 beginning at amino-acid T22 (ref.18). (f) IMR90s (G and S) were fractionated into chromatin-free (cytoplasmic plus nuclear soluble) and chromatin fractions and blotted with the indicated antibodies. Mek2 used as a cytoplasmic control and histones/H3 used as chromatin controls. (g) (Left) bioanalyzer trace of chromatin from G and S IMR90s upon MNase digestion and DNA isolation shows mononucleosomes. Mononucleosomes were blotted with the indicated antibodies to confirm presence of cleaved histone H3 products. (h) Immunoblots of growing and senescent (oncogene-induced and replicative senescence) melanocytes with the indicated antibodies (early, middle and late represent passages 4, 6 and 8, respectively). Asterisks indicate the proximal cleavage (cs2) and arrows indicate the distal cleavage (cs1). (i) Immunoblot of acid-extracted histones from primary growing melanocytes (mel) and fresh frozen human benign nevi samples (n=7) with αH3cs1. Figure 1: Histone H3 tail is processed upon oncogene-induced senescence in fibroblasts and melanocytes. ( a ) Inducible RAS V12 -driven OIS system in IMR90 fibroblasts evidenced by SA-β-Gal staining ( × 10 images shown), DAPI staining to monitor SAHF formation and EdU incorporation. Scale bars as shown. ( b ) Immunoblots of growing (G) and senescent (S) IMR90s with the indicated histone H3 PTM-specific antibodies. Asterisks indicate the proximal cleavage (cs2) and arrows indicate the distal cleavage (cs1). In all panels, core histones were stained with Amido Black for loading. ( c ) Immunoblot of the chromatin fraction of senescent IMR90s showing alignment of full-length and cleaved histone H3 products. H3cs1-specific antibody used for alignment of the distal cleavage product. ( d ) Diagram of histone H3 tail showing cleavage sites. Dashed lines indicate potential proximal cleavage (cs2) sites, as determined by immunoblotting with H3 PTM-specific antibodies. The solid line marks the distal cleavage site (cs1). ( e ) Immunoblot of growing and senescent IMR90 cells with a cleavage-specific antibody (αH3cs1), which recognizes the N terminus of H3 beginning at amino-acid T22 (ref. 18 ). ( f ) IMR90s (G and S) were fractionated into chromatin-free (cytoplasmic plus nuclear soluble) and chromatin fractions and blotted with the indicated antibodies. Mek2 used as a cytoplasmic control and histones/H3 used as chromatin controls. ( g ) (Left) bioanalyzer trace of chromatin from G and S IMR90s upon MNase digestion and DNA isolation shows mononucleosomes. Mononucleosomes were blotted with the indicated antibodies to confirm presence of cleaved histone H3 products. ( h ) Immunoblots of growing and senescent (oncogene-induced and replicative senescence) melanocytes with the indicated antibodies (early, middle and late represent passages 4, 6 and 8, respectively). Asterisks indicate the proximal cleavage (cs2) and arrows indicate the distal cleavage (cs1). ( i ) Immunoblot of acid-extracted histones from primary growing melanocytes (mel) and fresh frozen human benign nevi samples ( n =7) with αH3cs1. Full size image Using a combination of histone PTM-specific antibodies and an H3 cleavage-specific antibody (αH3cs1; ref. 18 ), we aligned the putative cleavage sites of the H3 tail ( Fig. 1c ). Because the H3K14ac antibody detects a faster migrating band that is not detectable with the H3K9me3 antibody, the proximal cleavage site most likely lies at or within the K9-K14 stretch (see Fig. 1d ). The distal cleavage site aligns with the H3cs1 antibody, which was designed to recognize H3 with a N terminus beginning at T22 ( Fig. 1c,d ; H3cs1 epitope: TKAAR [18] ). Therefore, we refer to the distal cleavage site as H3cs1 and the proximal site as H3cs2 ( Fig. 1d ). Owing to our ability to probe H3cs1 with a specific antibody, we focused our studies on this distal cleavage site. Levels of H3cs1 markedly increase upon OIS ( Fig. 1e ) and appear at much higher levels in senescent cells than mouse ESCs induced to differentiate ( Supplementary Fig. 2 ). We next investigated whether the cleaved H3 species were incorporated into chromatin and more specifically, nucleosomes. Growing and senescent IMR90s were fractionated into chromatin-free and chromatin fractions and probed with antibodies against H3cs1 and the C-terminal region of H3. Cleaved H3 products were detected only in the chromatin fraction of senescent cells ( Fig. 1f ). Next, soluble mononucleosomes were isolated from growing and senescent fibroblasts and immunoblotting revealed that cleaved H3 species are indeed nucleosomal in senescent cells ( Fig. 1g ). We highlight here that cleaved forms of the replication-independent histone variant H3.3 were also detected in these assays, suggesting that this histone variant may be preferentially processed in senescent cells (see below). Senescent melanocytes exhibit cleaved forms of H3 We also investigated chromatin changes in human primary melanocytes induced to senesce. These specialized pigment cells can remain senescent in human nevi (moles) for decades, and have the potential to progress into melanoma. We induced senescence via serial passaging of melanocytes (replicative senescence) and using the activated oncogene BRAF V600E (OIS) [6] . Senescence was monitored via multiple established assays ( Supplementary Fig. 3a–c ). As evidenced in Fig. 1h , the histone H3 tail is cleaved during both modes of senescence in primary human melanocytes. Interestingly, the same pattern of processing observed in fibroblasts is detected in melanocytes, and the fastest migrating species corresponds to H3cs1 ( Fig. 1h ). Like fibroblasts, the cleaved forms of H3 in senescent melanocytes are chromatin associated ( Supplementary Fig. 3d ). Next, we queried whether H3cs1 could be a marker of senescence in vivo by probing acid-extracted histones isolated from fresh frozen benign nevi for H3cs1. We identified the presence of H3cs1 in the majority of benign nevi samples tested (5/7), but not growing primary melanocytes ( Fig. 1i ). Further, by probing a panel of melanoma cell lines, we found that metastatic melanoma cells lack H3cs1, while primary melanoma lines that fail to proliferate in culture contain H3cs1 ( Supplementary Fig. 3e ). These findings suggest that H3cs1 may be a useful marker for assessing senescence in premalignant lesions. Processing of H3 requires activation of senescence programmes We questioned whether oncogene activation or DNA damage, in the absence of senescence, could trigger H3 cleavage. First, we examined cells subjected to oncogenic stress but unable to undergo senescence. E1A-transduced ER::H-RAS G12V IMR90s induced with 4OHT failed to enter senescence ( Supplementary Fig. 4a,b ), and were defective in H3 tail cleavage after 6 days of RAS G12V activation ( Supplementary Fig. 4c ). Moreover, acute induction of DNA damage via 24 h of etoposide treatment in IMR90s was not sufficient to induce H3 tail cleavage either ( Supplementary Fig. 4d ). Here, fibroblasts were arrested but not senescent as evidenced by various markers, including a lack of p16 expression ( Supplementary Fig. 4d,e ). These results strongly suggest that engagement of senescence effector pathways is required for the processing of H3. CTSL1 cleaves H3 and its inhibition impairs SAHF formation The lysosomal protease CTSL1 localizes to the nucleus upon RAS activation [20] and is responsible for cleaving the nuclear transcription factor CDP/Cux and the H3 tail [18] , [21] . To investigate whether CTSL1 is responsible for H3 tail cleavage during senescence, we first probed the levels of CTSL1 upon senescence induction in fibroblasts and melanocytes. CTSL1 levels increase transcriptionally and more strikingly at the protein level upon senescence in both systems ( Fig. 2a–c ). CTSL1 is found in three forms: the pro-cathepsin, intermediate and processed mature (active) forms [22] . Interestingly, our data show that the chromatin-bound pool of CTSL1 is enriched in the mature, active form of the protease, consistent with previous findings [18] . For example, at day 4 of senescence induction, only ~17% of CTSL1 exists in its mature form ( Fig. 2a ), while the chromatin-bound levels comprise ~40% ( Fig. 2b ). In senescent melanocytes, we could only detect the mature form of CTSL1 in the chromatin fraction ( Fig. 2c ). Finally, a detailed time-course analysis of the early stages of senescence in IMR90s demonstrates that CTSL1 messenger RNA expression correlates with detection of active CTSL1 in the chromatin fraction, precisely when H3 tail cleavage is observed ( Fig. 2b ). 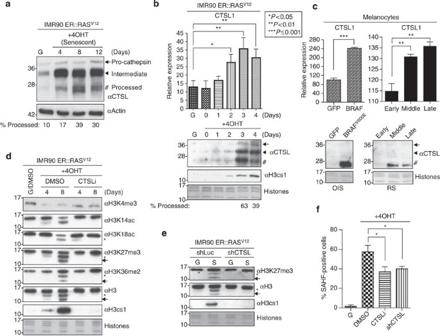Figure 2: Nuclear Cathepsin L mediates H3 tail processing and promotes SAHF. (a) Immunoblot for CTSL using whole-cell extract from growing and senescent IMR90s. Actin used for loading. (b) (Top) time course of CTSL1 induction as assessed by reverse transcription (RT)-quantitative (q)PCR. Values are normalized to expression of glyceraldehyde 3-phosphate dehydrogenase (GAPDH); mean±s.d. (n=3 biological replicates); two-tailed unpaired Student’st-test;Pvalues as indicated. (Bottom) immunoblot of the chromatin fraction from growing and senescent IMR90 cells with the indicated antibodies. In all panels, core histones were stained with Amido Black for loading. Samples for RT-qPCR and immunoblot analysis were obtained at identical time points. Note correlation of CTSL1 transcriptional induction, presence of the active form of CTSL1 in the chromatin fraction and H3 tail cleavage. (c) (Top) relative expression of CTSL1 in growing and senescent melanocytes assessed by RT-qPCR. Values are normalized to expression of GAPDH; mean±s.d. (n=3 technical replicates); two-tailed unpaired Student’st-test;Pvalues as indicated. (Bottom) immunoblot of CTSL using the chromatin fraction of growing and senescent melanocytes. (d) Chromatin extracts from growing and senescent IMR90 cells cultured in the presence of DMSO or a CTSL1 inhibitor probed with the indicated antibodies. Note the loss of H3 cleavage products in the CTSLi-treated cells, particularly at day 8. (e) Chromatin extracts from growing and senescent IMR90 cells expressing shLuc (control) or shCTSL1 lentiviral constructs probed with the indicated antibodies. Note the loss of H3 cleavage products in shCTSL1 senescent cells. (f) Quantification of SAHF in growing and senescent IMR90 cultured under the specified conditions obtained at day 8 post induction; mean±s.d. (n=3 biological replicates); two-tailed unpaired Student’st-test; DMSO versus CTSLi *P=0.0147; DMSO versus shCTSL *P=0.0147. Figure 2: Nuclear Cathepsin L mediates H3 tail processing and promotes SAHF. ( a ) Immunoblot for CTSL using whole-cell extract from growing and senescent IMR90s. Actin used for loading. ( b ) (Top) time course of CTSL1 induction as assessed by reverse transcription (RT)-quantitative (q)PCR. Values are normalized to expression of glyceraldehyde 3-phosphate dehydrogenase (GAPDH); mean±s.d. ( n =3 biological replicates); two-tailed unpaired Student’s t -test; P values as indicated. (Bottom) immunoblot of the chromatin fraction from growing and senescent IMR90 cells with the indicated antibodies. In all panels, core histones were stained with Amido Black for loading. Samples for RT-qPCR and immunoblot analysis were obtained at identical time points. Note correlation of CTSL1 transcriptional induction, presence of the active form of CTSL1 in the chromatin fraction and H3 tail cleavage. ( c ) (Top) relative expression of CTSL1 in growing and senescent melanocytes assessed by RT-qPCR. Values are normalized to expression of GAPDH; mean±s.d. ( n =3 technical replicates); two-tailed unpaired Student’s t -test; P values as indicated. (Bottom) immunoblot of CTSL using the chromatin fraction of growing and senescent melanocytes. ( d ) Chromatin extracts from growing and senescent IMR90 cells cultured in the presence of DMSO or a CTSL1 inhibitor probed with the indicated antibodies. Note the loss of H3 cleavage products in the CTSLi-treated cells, particularly at day 8. ( e ) Chromatin extracts from growing and senescent IMR90 cells expressing shLuc (control) or shCTSL1 lentiviral constructs probed with the indicated antibodies. Note the loss of H3 cleavage products in shCTSL1 senescent cells. ( f ) Quantification of SAHF in growing and senescent IMR90 cultured under the specified conditions obtained at day 8 post induction; mean±s.d. ( n =3 biological replicates); two-tailed unpaired Student’s t -test; DMSO versus CTSLi * P =0.0147; DMSO versus shCTSL * P =0.0147. Full size image Next, we used both chemical inhibition (CTSLi) and short hairpin RNA (shRNA) approaches to assess the role of CTSL1 in processing the H3 tail. IMR90 ER::RAS V12 cells were induced to senesce with 4OHT in the presence of either dimethyl sulfoxide (DMSO) or a potent irreversible CTSL1-specific inhibitor ( Fig. 2d ). This inhibitor blocks self-processing of CTSL1 into its mature form, leading to the accumulation of the intermediate form ( Supplementary Fig. 5a ). In addition, ER::RAS V12 -infected fibroblasts were engineered to express either shCTSL1 or shLuc control. This knockdown was specific for CTSL1 and was maintained over a 2-week course of senescence ( Supplementary Fig. 5 ). In both scenarios, when cells were induced to senesce, we observed a block in the production of both H3cs1 and cs2 ( Fig. 2d,e ). This implicates CTSL1 as the key protease responsible for the observed cleavage events. Of note, we observed that loss of H3K4me3 is less pronounced upon CTSL inhibition as compared with DMSO-treated cells ( Fig. 2d , and see below). In addition, we queried whether CTSL1 inhibition, and thus a block in H3 cleavage, could bypass OIS. The inhibition of CTSL1 did not allow for increased proliferation in IMR90 ER::RAS V12 cells induced to senesce ( Supplementary Fig. 6 ), however, its inhibition/deficiency significantly impaired SAHF formation ( Fig. 2f ). While these data show that CTSL1 inhibition alone is not sufficient to bypass a robust senescence system such as RAS V12 -driven OIS in IMR90s, they do suggest that CTSL1 activity and its downstream substrates (H3 and possibly others) are important for SAHF formation. H3.3 and H3.3cs1 induce a senescence programme Canonical H3.1 and the variant H3.3 differ by only five amino acids. Four of these residues cluster in the interface between H3.3 and H4, a region that mediates the interaction with distinct histone chaperone complexes [23] . The other differential amino acid is at position 31, which resides in the histone tail ( Fig. 1d ). To assess which H3 isoform is proteolytically processed during senescence, we first probed the chromatin fraction of growing and senescent cells with an antibody against H3.3 (which recognizes the C terminus of the histone). We verified this antibody is specific for H3.3 by immunoblotting tagged forms of H3.1 and H3.3 ( Supplementary Fig. 7a ). Using this antibody, we detected H3.3 cleavage products in senescent fibroblasts and melanocytes ( Fig. 1f ; Supplementary Fig. 4d ). Moreover, H3.3 and its cleavage products are incorporated into nucleosomes ( Fig. 1g ). As previously reported [10] , we also find increased levels of H3.3 during a senescence time course ( Supplementary Fig. 7b ). Next, we inquired whether ectopic expression of full-length forms of Flag-tagged H3.1 (H3.1FL) and H3.3 (H3.3FL) could induce senescence in IMR90s. As expected, these ectopically expressed histones are localized to the nucleus by immunofluorescence ( Supplementary Fig. 7c ). Intriguingly, by immunoblotting for Flag, we observed that H3.3 is cleaved with a similar pattern to that of OIS ( Fig. 3a,b ). Because of this finding, we next inquired whether expression of H3.3FL or H3.3cs1 was sufficient to induce senescence in IMR90s in the absence of oncogenic signalling. Thus, we generated H3.3cs1-Flag, which co-migrates with the faster migrating band of H3.3FL-Flag-cleavage products ( Fig. 3b ). Further supporting our investigation of H3.3cs1 in senescence, the identical construct generated for H3.1 (H3.1cs1) was not expressed or incorporated into chromatin ( Supplementary Fig. 7c,d ), suggesting that histone chaperone recognition was compromised or that this form of H3.1 may not be physiologically relevant. 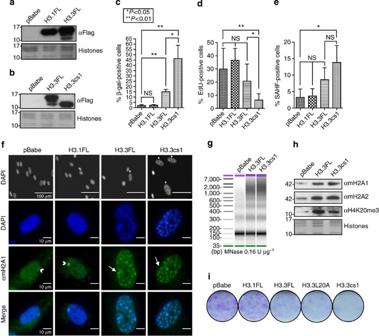Figure 3: Ectopic expression of H3.3 and H3.3cs1 induces senescence in fibroblasts. (a,b) Immunoblot of IMR90 cells stably expressing full-length H3.1 (H3.1FL), full-length H3.3 (H3.3FL), cleaved H3.3 (H3.3cs1) or empty pBabe vector with αFlag. Core histones stained with Amido Black for loading. Note the H3 cleavage products in H3.3FL-expressing cells. (c) Quantification of β-Gal-positive cells in IMR90 cells expressing the indicated histones; mean±s.d. (n=3 biological replicates). (d) Quantification of EdU incorporation; mean±s.d. (n=3 biological replicates). (e) Quantification of SAHF; mean±s.d. (n=3 biological replicates);Pvalues forc–eare as indicated; two-tailed unpaired Student’st-test. (f) (Top) DAPI-stained nuclei of IMR90s expressing the indicated histones. Scale bars as shown. (Middle) immunofluorescence of IMR90s expressing the indicated histones stained with DAPI and αmacroH2A1. Arrowheads indicate Xi and arrows indicate SAHF. (Bottom). Merged images of DAPI and αmacroH2A1. Images taken at × 40 magnification. (g) Nuclei obtained from IMR90s expressing the indicated histones were digested with MNase at 0.16 units per μg of chromatin. DNA was isolated after MNase digestion and analysed by a high-sensitivity DNA assay (Agilent 2100 Bioanalyzer). (h) Chromatin fraction from IMR90 cells expressing pBabe, H3.3FL and H3.3cs1 probed with the indicated antibodies. Core histones stained with Amido Black for loading. (i) Colony formation assay course (day 16 post infection) of IMR90s expressing the indicated histones. NS, not significant. Figure 3: Ectopic expression of H3.3 and H3.3cs1 induces senescence in fibroblasts. ( a , b ) Immunoblot of IMR90 cells stably expressing full-length H3.1 (H3.1FL), full-length H3.3 (H3.3FL), cleaved H3.3 (H3.3cs1) or empty pBabe vector with αFlag. Core histones stained with Amido Black for loading. Note the H3 cleavage products in H3.3FL-expressing cells. ( c ) Quantification of β-Gal-positive cells in IMR90 cells expressing the indicated histones; mean±s.d. ( n =3 biological replicates). ( d ) Quantification of EdU incorporation; mean±s.d. ( n =3 biological replicates). ( e ) Quantification of SAHF; mean±s.d. ( n =3 biological replicates); P values for c – e are as indicated; two-tailed unpaired Student’s t -test. ( f ) (Top) DAPI-stained nuclei of IMR90s expressing the indicated histones. Scale bars as shown. (Middle) immunofluorescence of IMR90s expressing the indicated histones stained with DAPI and αmacroH2A1. Arrowheads indicate Xi and arrows indicate SAHF. (Bottom). Merged images of DAPI and αmacroH2A1. Images taken at × 40 magnification. ( g ) Nuclei obtained from IMR90s expressing the indicated histones were digested with MNase at 0.16 units per μg of chromatin. DNA was isolated after MNase digestion and analysed by a high-sensitivity DNA assay (Agilent 2100 Bioanalyzer). ( h ) Chromatin fraction from IMR90 cells expressing pBabe, H3.3FL and H3.3cs1 probed with the indicated antibodies. Core histones stained with Amido Black for loading. ( i ) Colony formation assay course (day 16 post infection) of IMR90s expressing the indicated histones. NS, not significant. Full size image Through a rigorous series of experiments, we found that H3.3cs1 induces senescence in fibroblasts compared with empty vector control (pBabe) and H3.1FL. Importantly, ectopic H3.3cs1 is expressed at similar levels to that of endogenous H3cs1 during OIS ( Supplementary Fig. 8a ). H3.3FL can also induce senescence, albeit in a less robust manner than H3.3cs1. Senescence induction in this system was monitored by cell morphology and SA-β-gal staining ( Fig. 3c ), incorporation of EdU to assess DNA replication ( Fig. 3d ), expression of CCNA (Cyclin A2), p16, p21 ( Supplementary Fig. 8b–d ) and SAHF formation ( Fig. 3e ). Consistent with a senescent phenotype, cells expressing H3.3FL and H3.3cs1 showed larger nuclei than those expressing H3.1FL or pBabe ( Fig. 3f , top panel). At higher magnification, DAPI-dense SAHFs were clearly observed only in H3.3FL- and H3.3cs1-expressing fibroblasts ( Fig. 3f ). Moreover, these SAHFs stained positively for macroH2A1, a late marker of SAHF formation [12] , suggestive of established SAHFs ( Fig. 3f ). Further, we find that H3.3FL and H3.3cs1 induce heterochromatization as evidenced by increased resistance to digestion with micrococcal nuclease ( Fig. 3g ) and changes in the PTM and histone variant profile consistent with senescence, including increased H4K20me3 and macroH2A levels ( Fig. 3h ). Next we questioned whether H3.3L20A, a mutation of H3 that prevents CTSL1-mediated cleavage [24] , would induce senescence. Colony formation assays ( Fig. 3i ), quantitation of SA-β-gal staining and incorporation of EdU ( Supplementary Fig. 9 ) showed that L20A induces a senescence phenotype similar to that of wild-type H3.3FL. These findings suggest that full-length H3.3 indeed plays a role in senescence independent of its proteolytic processing, which is not unexpected as senescent cells rely on DNA replication-independent incorporation of histone H3.3 as they exit the cell cycle [25] . Taken together, these results provide evidence that the predominant form of H3 proteolytically processed by CTSL1 during senescence is H3.3. Moreover, they demonstrate that H3.3 and more robustly its cleaved product (H3.3cs1), but not H3.1, can drive a cellular senescence programme. HUCA is required for chromatin incorporation of H3.3cs1 Next, we examined the localization of Flag-tagged H3.3FL and H3.3cs1 in IMR90s. H3.3FL and H3.3cs1 were found largely excluded from SAHF, which were marked by H3K9me3 ( Fig. 4a ). This is consistent with a recent study that also showed exclusion of H3.3 from SAHF [25] . These data further suggest that cleavage of H3.3 does not compromise H3K9me3, which is likely to be found on canonical H3.1 or H3.2 in SAHF. 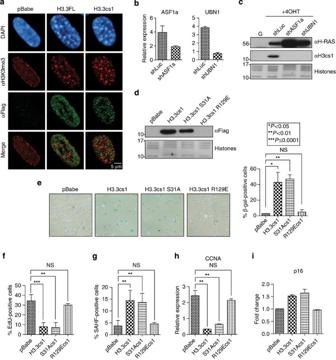Figure 4: The histone chaperone complex HUCA is required for chromatin incorporation of H3.3cs1. (a) Confocal microscopy of Flag-tagged H3.3FL and H3.3cs1. DAPI, H3K9me3 (red), Flag (green) staining and merged (red and green) images shown. (b) Confirmation of ASF1a and UBN1 knockdown in IMR90 ER::RASV12cells by reverse transcription-quantitative PCR. Values are normalized to expression of glyceraldehyde 3-phosphate dehydrogenase (GAPDH); mean±s.d. (n=2 biological replicates for ASF1a andn=3 technical replicates for UBN1). (c) Chromatin fraction from growing and senescent IMR90 ER::RASV12cells expressing either shLuc, shASF1a or shUBN1 probed with αH3cs1. αH-RAS immunoblot shows inducible expression of RASV12. Core histones stained with Amido Black for loading. (d) Immunoblot of the chromatin fraction of IMR90 cells expressing the indicated histones with αFlag. (e) Representative SA-β-Gal staining images of IMR90 expressing the indicated histones ( × 10 images shown); quantification shown on the right; mean±s.d. (n=2 biological replicates with three technical replicates). (f–i) Quantification of EdU incorporation, SAHF-positive cells, CCNA and p16 levels in IMR90 cells expressing the indicated histones. Values are normalized to expression of GAPDH; mean±s.d. (n=3 technical replicates);Pvalues fore–ias indicated; two-tailed unpaired Student’st-test. For p16, expression is relative to pBabe control. NS, not significant. Figure 4: The histone chaperone complex HUCA is required for chromatin incorporation of H3.3cs1. ( a ) Confocal microscopy of Flag-tagged H3.3FL and H3.3cs1. DAPI, H3K9me3 (red), Flag (green) staining and merged (red and green) images shown. ( b ) Confirmation of ASF1a and UBN1 knockdown in IMR90 ER::RAS V12 cells by reverse transcription-quantitative PCR. Values are normalized to expression of glyceraldehyde 3-phosphate dehydrogenase (GAPDH); mean±s.d. ( n =2 biological replicates for ASF1a and n =3 technical replicates for UBN1). ( c ) Chromatin fraction from growing and senescent IMR90 ER::RAS V12 cells expressing either shLuc, shASF1a or shUBN1 probed with αH3cs1. αH-RAS immunoblot shows inducible expression of RAS V12 . Core histones stained with Amido Black for loading. ( d ) Immunoblot of the chromatin fraction of IMR90 cells expressing the indicated histones with αFlag. ( e ) Representative SA-β-Gal staining images of IMR90 expressing the indicated histones ( × 10 images shown); quantification shown on the right; mean±s.d. ( n =2 biological replicates with three technical replicates). ( f – i ) Quantification of EdU incorporation, SAHF-positive cells, CCNA and p16 levels in IMR90 cells expressing the indicated histones. Values are normalized to expression of GAPDH; mean±s.d. ( n =3 technical replicates); P values for e – i as indicated; two-tailed unpaired Student’s t -test. For p16, expression is relative to pBabe control. NS, not significant. Full size image Because the ectopic expression of H3.3FL and H3.3cs1 demonstrated a largely euchromatic nuclear localization ( Fig. 4a ), we hypothesized that the HUCA histone chaperone complex may be responsible for H3.3cs1 deposition in senescent cells. The HUCA histone chaperone complex interacts specifically with H3.3, and is responsible for its deposition at distinct chromatin regions, including transcription start sites and the bodies of active genes [26] , [27] . To test whether this complex is required for chromatin incorporation of endogenous H3cs1 during OIS senescence, IMR90 ER::RAS V12 cells were infected with lentiviral shRNAs against HIRA, ASF1a, UBN1 or luciferase control and induced to senesce. During the course of these studies, we noted that the HIRA knockdown was reproducibly incompatible with cell viability, and we therefore focused on knockdown of ASF1a and UBN1. Upon knockdown of either ASF1a or UBN1 ( Fig. 4b ; Supplementary Fig. 10a ), we observed a marked reduction in the incorporation of H3cs1 in the chromatin fraction compared with control cells ( Fig. 4c ). This was specific for HUCA, as knockdown of Daxx, a component of a separate chaperone that deposits H3.3 at telomeres [28] , [29] , did not affect H3cs1 levels in chromatin ( Supplementary Fig. 10b,c ). To complement these findings, we investigated whether ASF1a mediates the ability of ectopically expressed H3.3cs1 to induce senescence in IMR90s in the absence of oncogenic signalling. We generated an H3.3cs1-Flag construct with an R-to-E substitution at position 129 (R129E), a mutation that has been shown to disrupt interaction of H3.3 with ASF1a (ref. 23 ). We also generated H3.3cs1-Flag containing an S-to-A substitution at position 31 (S31A), which mimics the tail of H3.1 and is not likely to alter chaperone binding. IMR90 cells were transduced with pBabe, H3.3cs1, H3.3cs1 S31A and H3.3cs1 R129E ( Fig. 4d ). Immunoblots with α-Flag demonstrate that while H3.3cs1 and H3.3cs1 S31A are incorporated into chromatin, H3.3cs1 R129E is not ( Fig. 4d ). Consistent with these findings, H3.3cs1 S31A induces senescence as efficiently as H3.3cs1, as measured by changes in cell morphology and increased SA-β-gal staining ( Fig. 4e ), loss of EdU incorporation ( Fig. 4f ), induction of SAHF formation ( Fig. 4g ), decreased CCNA expression ( Fig. 4h ) and induction of p16 ( Fig. 4i ). On the other hand, H3.3cs1 R129E failed to induce senescence markers in IMR90 cells by all accounts ( Fig. 4e–i ). Collectively, these data suggest that ASF1a and UBN1, via direct interaction with H3.3, are required for incorporation of cleaved H3.3 into chromatin. H3.3cs1 represses E2F target genes via H3K4me3 loss To gain a better understanding of the gene expression programme mediated by cleaved H3.3, we performed RNA-seq of growing and OIS fibroblasts, as well as fibroblasts expressing H3.3cs1 at two different time points post infection (early: day 3 and late: day 13). As expected, we found a marked change in the gene expression programme of OIS as compared with growing cells ( Fig. 5a ; Supplementary Table 1 ). Interestingly, we noted that the majority of the differentially expressed genes in the H3.3cs1-induced senescence samples at both early and late time points were downregulated when compared with growing cells. We found a striking significant overlap between these downregulated genes and genes downregulated in OIS ( Fig. 5a,b ), suggesting that similar pathways are repressed in both systems. Consistent with our previous findings [15] , Gene Ontology (GO) analysis reveals that OIS and H3.3cs1-downregulated genes are similarly involved in cell cycle progression ( Supplementary Fig. 11a ). To understand transcription factor enrichment for the differentially expressed downregulated genes during both OIS and H3.3cs1-induced senescence, we used the ChIP-X Enrichment Analysis tool (ChEA), which contains gene lists for 205 different mammalian transcription factors extracted from over 230 chromatin immunoprecipitation-sequencing (ChIP-seq) or ChIP-chip publications [30] . This analysis confirms that these downregulated genes are targets of a common set of transcription factors and epigenetic regulators, including members of the E2F family and the H3K4me3 demethylase KDM5B (JARID1B) ( Fig. 5c ). 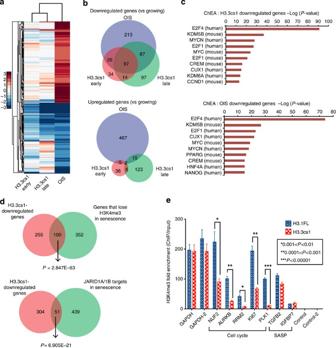Figure 5: H3.3cs1-induced senescence is mediated by decreased transcriptional output of cell cycle genes and reduced H3K4me3. (a) Heat map showing gene expression changes of 914 genes as determined by RNA-seq in H3.3cs1-induced senescence (early and late time points) relative to those that are altered in OIS (versus growing). Note the overlap of downregulated genes between H3.3cs1-induced senescence and OIS. (b) (Top) venn diagram of genes downregulated in OIS, H3.3cs1 (early) and H3.3cs1 (late) as compared with growing IMR90s. Fisher exact test;P=2.418E−117 OIS versus H3.3cs1 (early);P=3.477E−162 OIS versus H3.3cs1 (late);P=2.404E−117 H3.3cs1 (early) versus H3.3cs1 (late). (Bottom) venn diagram of genes upregulated in OIS, H3.3cs1 (early) and H3.3cs1 (late) as compared with growing IMR90s. Fisher exact test;P=3.414E−4 OIS versus H3.3cs1 (early);P=2.883E−7 OIS versus H3.3cs1 (late);P=1.783E−7 H3.3cs1 (early) versus H3.3cs1 (late). (c) ChIP Enrichment Analysis (ChEA) of H3.3cs1-induced senescence (top) and OIS (bottom)-downregulated genes. Note that E2F family members and KDM5B (JARID1B) gene targets are enriched in both. The −log of thePvalue associated with each term is plotted. (d) Venn diagrams illustrating the overlap between H3.3cs1-downregulated genes and genes that lose H3K4me3 in senescence and JARID1A/1B-regulated genes in senescence15. Fisher exact test ofPvalues indicated in the diagram. (e) ChIP-quantitative PCR for H3K4me3 at cell cycle genes and SASP-related genes in IMR90s expressing H3.1FL (blue) or H3.3cs1 (red). Two regions near the glyceraldehyde 3-phosphate dehydrogenase (GAPDH) promoter used as positive controls; intergenic regions used as negative controls. Fold enrichment of H3K4me3 ChIP/input is plotted. Mean±s.e.m.; two-tailed paired samplet-test;Pvalues as indicated. Figure 5: H3.3cs1-induced senescence is mediated by decreased transcriptional output of cell cycle genes and reduced H3K4me3. ( a ) Heat map showing gene expression changes of 914 genes as determined by RNA-seq in H3.3cs1-induced senescence (early and late time points) relative to those that are altered in OIS (versus growing). Note the overlap of downregulated genes between H3.3cs1-induced senescence and OIS. ( b ) (Top) venn diagram of genes downregulated in OIS, H3.3cs1 (early) and H3.3cs1 (late) as compared with growing IMR90s. Fisher exact test; P =2.418E−117 OIS versus H3.3cs1 (early); P =3.477E−162 OIS versus H3.3cs1 (late); P =2.404E−117 H3.3cs1 (early) versus H3.3cs1 (late). (Bottom) venn diagram of genes upregulated in OIS, H3.3cs1 (early) and H3.3cs1 (late) as compared with growing IMR90s. Fisher exact test; P =3.414E−4 OIS versus H3.3cs1 (early); P =2.883E−7 OIS versus H3.3cs1 (late); P =1.783E−7 H3.3cs1 (early) versus H3.3cs1 (late). ( c ) ChIP Enrichment Analysis (ChEA) of H3.3cs1-induced senescence (top) and OIS (bottom)-downregulated genes. Note that E2F family members and KDM5B (JARID1B) gene targets are enriched in both. The −log of the P value associated with each term is plotted. ( d ) Venn diagrams illustrating the overlap between H3.3cs1-downregulated genes and genes that lose H3K4me3 in senescence and JARID1A/1B-regulated genes in senescence [15] . Fisher exact test of P values indicated in the diagram. ( e ) ChIP-quantitative PCR for H3K4me3 at cell cycle genes and SASP-related genes in IMR90s expressing H3.1FL (blue) or H3.3cs1 (red). Two regions near the glyceraldehyde 3-phosphate dehydrogenase (GAPDH) promoter used as positive controls; intergenic regions used as negative controls. Fold enrichment of H3K4me3 ChIP/input is plotted. Mean±s.e.m. ; two-tailed paired sample t -test; P values as indicated. Full size image Previously, we reported that RB and JARID1A/1B cooperate in the silencing of E2F targets during senescence via H3K4me3 demethylation [15] . To investigate a potential role for H3 tail cleavage in the removal of H3K4me3, we compared our RNA-seq results with the ChIP-seq and gene expression data from that study. We found a significant overlap between H3.3cs1-downregulated genes and those genes in which H3K4me3 is lost during senescence ( Fig. 5d , top). Furthermore, the overlap between H3.3cs1-downregulated genes and those regulated by JARID1A/1B ( Fig. 5d , bottom) and RB ( Supplementary Fig. 11b ) is highly significant. Next, we performed ChIP for H3K4me3 in IMR90s expressing either H3.1FL (which does not induce senescence) or H3.3cs1 (which induces senescence). We focused on the promoters of representative cell cycle-promoting genes, senescence-associated secretory phenotype (SASP)-related genes (see below), glyceraldehyde 3-phosphate dehydrogenase (not transcriptionally altered upon senescence), as well as intergenic regions that are not occupied by H3K4me3 as negative controls ( Fig. 5e ). We found that cell cycle genes that are transcriptionally downregulated during H3.3cs1-induced senescence (via RNA-seq) show significantly less H3K4me3 at their promoters as compared with H3.1FL-expressing cells. Of note, these representative genes are also downregulated in OIS, but are not reported targets of the JARID1A/1B demethylases [15] . Together, these data support a model in which H3.3 tail cleavage functions in a similar manner as the JARID1 demethylases to remove H3K4me3 and facilitate silencing of proliferation-promoting RB/E2F target genes during senescence ( Fig. 6 ). It further suggests that the proteolytic processing of the H3.3 tail functions as a key mechanism for H3K4me3 loss at a subset of genes that are downregulated during senescence. This is supported by the fact that CTSL inhibition partially impedes the loss of H3K4me3 in senescent cells ( Fig. 2d , top blot). 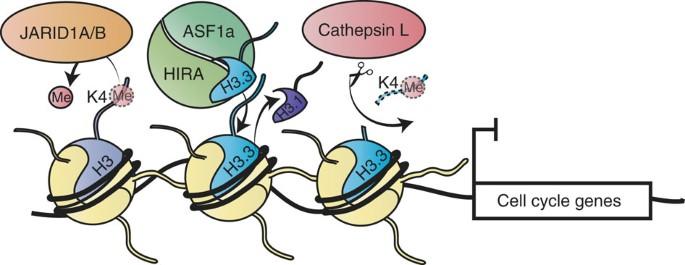Figure 6: Model depicting the mechanisms of H3K4me3 loss in senescence. The HUCA histone chaperone complex showing ASF1a/HIRA is depicted depositing H3.3, coupled to eviction of replication-dependent histone H3.1. Both JARID1A/1B-mediated demethylation and CTSL-mediated proteolytic processing of H3.3 tail act to prevent transcription of cell cycle-related genes via removal of H3K4me3. These processes may work together or independently to ensure the silencing of proliferation-promoting genes during cellular senescence. Figure 6: Model depicting the mechanisms of H3K4me3 loss in senescence. The HUCA histone chaperone complex showing ASF1a/HIRA is depicted depositing H3.3, coupled to eviction of replication-dependent histone H3.1. Both JARID1A/1B-mediated demethylation and CTSL-mediated proteolytic processing of H3.3 tail act to prevent transcription of cell cycle-related genes via removal of H3K4me3. These processes may work together or independently to ensure the silencing of proliferation-promoting genes during cellular senescence. Full size image Finally, we observed that a much larger set of genes is upregulated during OIS than during H3.3cs1-induced senescence (early and late) compared with growing cells ( Fig. 5a ), and that there is little overlap between these groups ( Fig. 5b , bottom). GO analysis of the upregulated genes in each system reveals that in fact different biological processes are affected ( Supplementary Fig. 11c,d ). Fibroblasts undergoing OIS display induction of cell signalling, inflammatory and secretory pathways that play a major role in the SASP [7] , [31] , [32] . This includes interleukin 6, interleukin 8, matrix metalloproteinase 3 and CXCL1, among others (see Supplementary Table 1 ). Interestingly, H3.3cs1-induced senescence appears largely deficient in SASP induction, which may explain in part the milder senescence phenotype observed as compared with RAS V12 -induced senescence. We note, however, that some SASP-like factors such as IGFBP2, 3, 7 and transforming growth factorβ2 were induced upon H3.3cs1 ectopic expression. While heterogeneous in nature, multiple lines of evidence suggest that a persistent DNA damage response is required to trigger SASP [32] , [33] . Consistent with this, we found that while OIS triggers a DNA-damage response as previously reported [34] , [35] , H3.3cs1 overexpression fails to do so ( Supplementary Fig. 12 ). Although senescence is associated with marked reorganization of chromatin structure, the distinct mechanistic chromatin-mediated events that contribute to this process remain poorly understood. Here we uncover novel senescence-associated proteolytic processing of histone H3 mediated by CTSL1 in human fibroblasts and melanocytes. CTSL1 cleaves the histone H3 tail at least at two distinct sites generating new N termini at residues T22 (H3cs1), as previously reported in differentiating mouse ESCs [18] , and a novel site likely between K9 and K14 (H3cs2). Of note, H3cs2 was not identified in ESCs upon differentiation [18] , and thus appears specific for cellular senescence. It will be of interest in the future to map the precise N terminus of H3cs2, determine whether the cs1 and cs2 cleavage events occur sequentially or simultaneously and to investigate whether H3cs2 can also induce senescence. Recently, a study showed evidence of senescence-associated H3 tail cleavage, however, this was reported to be a cytoplasmic event [36] . In that study, H3 tail processing was due to chromatin fragments budding out of the nucleus as a consequence of disrupted nuclear envelope integrity. In turn, histones could be processed by lysosomes and progressively depleted. We have no evidence to suggest cytoplasmic processing of H3 in our systems and demonstrate that cleaved forms of H3 are indeed associated with chromatin and incorporated into nucleosomes. Moreover, the presence of active CTSL1 in the chromatin fraction of senescent cells is consistent with findings from other systems [18] , [20] , [21] , [37] . However, it remains plausible that a small fraction of cytoplasmic H3cs1 was not detectable by our biochemical methods or that the appearance of such cytoplasmic histone processing occurs at later time points of senescence than we have assayed. Because H3.3 is deposited into chromatin in a DNA replication-independent manner, it is likely that non-dividing cells, such as those undergoing senescence, depend on incorporation of H3.3. In fact, a recent study shows that while newly synthesized H3.3 is actively deposited into chromatin of senescent cells, H3.1 is not [25] . Consistent with this idea, we and others have found increased levels of H3.3 in the chromatin template of senescent cells ( Supplementary Fig. 7b ; reviewed in ref. 10 ). We also found that the ectopic expression of H3.3, but not H3.1, induces a senescence programme in fibroblasts characterized by classic markers of bona fide senescence, including increased SA-β-Gal activity and formation of macroH2A-containing SAHF ( Fig. 3 ). The observed senescence phenotype is more robust with cleaved H3.3 (H3.3cs1) than the full-length histone, suggesting that the proteolytic processing of H3.3 is particularly important. The fact that the ASF1a and UBN1 are required for the chromatin incorporation of H3cs1 during senescence is consistent with studies reporting a role for HIRA and ASF1a in senescence [12] . We further demonstrate that the ability of ectopic H3.3cs1 to induce senescence is dependent on its ability to directly interact with ASF1a ( Fig. 4 ). Because HIRA knockdown is incompatible with fibroblast viability, we cannot exclude a role for HIRA in H3.3cs1 deposition, and suggest that it may play distinct roles in proliferating versus senescent cells. Interestingly, while histone chaperone complexes have preferred histone targets (for example, HUCA with H3.3 and HJURP with CENPA), evidence to date suggests that upon altered cellular conditions, alternate chaperone complexes can deposit histones if the preferred factor is not available or the histone is overexpressed [27] , [28] , [38] . However, our data suggest that HUCA is unique in its ability to incorporate H3.3cs1 into chromatin, as other chaperones could not compensate in its absence or for a disruption of the H3.3–ASF1a interaction in IMR90 cells. While HUCA components HIRA and ASF1a have been implicated in regulating senescence [12] , [39] , our studies suggest for the first time that their substrate H3.3, as well as its nucleosome-incorporated cleaved product H3.3cs1, play an important role in promoting senescence. Consistent with data from others [25] , our immunofluorescence data suggest that H3.3 is largely excluded from SAHF. Interestingly, we also show that CTSL1 inhibition/knockdown leads to defective SAHF formation during OIS, raising the possibility that H3 tail cleavage may play a role in the reorganization of chromatin during senescence. Here, we provide evidence that H3.3cs1 can mediate gene expression pathways consistent with senescence. Specifically, we found that H3.3cs1 mediates the transcriptional repression of a large subset of genes previously shown to be downregulated by RB and JARID1A/1B during senescence [15] . Similar to RB- and JARID1-regulated genes, a large subset of H3.3cs1-downregulated genes lose H3K4me3 and are primarily E2F targets involved in cell cycle progression. We find that such transcriptional suppression occurs even at very early time points after introduction of H3.3cs1 (for example, 3 days; Fig. 5a,b ), and is coupled to a lack of H3K4me3 promoter occupancy ( Fig. 5e ), suggesting that these genes may be direct targets of the cleaved histone. Finally, we propose that HUCA incorporates H3.3 during senescence in a replication-independent manner, likely replacing H3.1 at genomic locations including the promoter or regulatory regions of cell cycle-promoting genes ( Fig. 6 ). JARID1A/1B-mediated demethylation and CTSL1-mediated H3.3 tail cleavage may cooperate or work independently in the removal of H3K4me3, thus contributing to the transcriptional suppression of these genes ( Fig. 6 ). Owing to the significant overlap between JARID1A/1B and H3.3cs1 target genes, histone demethylation and cleavage mechanisms may act synergistically at neighbouring nucleosomes or at the very same nucleosomes. Furthermore, because H3 tail cleavage is a more stable chromatin modification than enzymatic demethylation, the removal of H3K4me3 via histone proteolysis may contribute to long-term repression of proliferation-promoting genes and thus, the irreversible nature of senescence. Collectively, our studies have identified a novel biological function for the proteolytic cleavage of H3.3 in senescence, and we look forward to studies that characterize the cleavage of H3 and other histones/histone variants in their respective biological contexts. Cell culture IMR90 fibroblasts were grown in Dulbecco's modified Eagle's medium supplemented with 10% foetal bovine serum and 1% penicillin/streptomycin. Normal human melanocytes were isolated from the epidermis of neonatal foreskins and cultured in Melanocyte Growth Media 254 supplemented with Human Melanocyte Growth Supplement (Life Technologies). Plasmids and shRNA The following retroviral and lentiviral constructs were used in this study: pLNCX2-neo (ER::RAS V12 ) [19] , HIV-CS-CGBRAFE600-puro and pLL3.7-GFP (Addgene). Human full-length and cleaved histone H3 constructs were cloned into the retroviral vector pBabe-puro (Addgene) with a C-terminal Flag tag and expressed in IMR90 cells. Point mutations of H3.3cs1 were synthesized by Invitrogen (GeneArt) and subsequently cloned into the pBabe vector (BamHI-EcoRI). For shRNA studies, IMR90 cells were infected with lentiviral constructs encoding CTSL1 shRNAs (Open Biosystems, RHS4533-NM_001912), ASF1a shRNA (The RNAi Consortium validated TRCN0000074269), shDaxx (TRCN0000003800), shUBN1 (TRCN0000017813) or luciferase shRNA by standard procedures. Infected cells were selected using either 1 μg ml −1 puromycin or 800 μg ml −1 neomycin. OIS OIS was performed as described [19] . Briefly, IMR90 human diploid fibroblasts were transduced with a tamoxifen-inducible H-RAS V12 construct (pLNCX2-neo ER::RAS V12 ). A final concentration of 100 nM 4OHT was used to induce senescence over a 2-week period. Senescence induction with BRAF V600E in melanocytes was performed as described [6] . Briefly, human neonatal primary melanocytes (passage 2) were transduced with the lentiviral constructs HIV-CS-CGBRAFE600-puro or pLL3.7-GFP control. BRAFV600E-expressing cells were selected with puromycin at 1 μg ml −1 for 3–4 days and grown in supplemented Melanocyte Growth Media 254 for a total of 21 days post infection. CTSL1 inhibition For CTSL1 inhibition studies, IMR90 ER::RAS V12 cells were cultured under growing conditions or induced to senesce with 100 nM 4OHT in the presence of either DMSO or 1–5 μM CTSL1 inhibitor (Calbiochem, 219421-1MG). Chromatin fractionation and histone acid extraction Chromatin fractionation was performed as described [40] . Briefly, cell pellets were resuspended in buffer A (10 mM Hepes pH=7.9, 10 mM KCl, 1.5 mM MgCl 2 , 0.34 M sucrose, 10% glycerol, 0.1% triton-X, supplemented with protease inhibitor cocktail (Calbiochem, 539131) and 1 mM dithiothreitol (DTT)) and incubated on ice for 7–8 min. Nuclei were harvested by centrifugation at 4,000 r.p.m. for 5 min, and the supernatant containing the cytoplasmic fraction was collected. Pelleted nuclei were washed once with triton-free Buffer A before incubation in no-salt buffer (3 mM EDTA, 0.2 mM EGTA, 1 mM DTT and protease inhibitor) on ice for 40 min. The chromatin fraction was recovered by centrifugation at 4,000 r.p.m. for 5 min. Supernatant from this last step containing the nuclear-soluble fraction was mixed with the cytoplasmic fraction to obtain the chromatin-free fraction. Histone acid extraction was performed as described [41] . Briefly, fresh frozen nevi were ground in hypotonic lysis buffer (10 mM Tris–HCl pH 8.0, 1 mM KCl, 1.5 mM MgCl 2 , 0.5% NP-40, 1 mM DTT, protease inhibitors), lysed for 30 min on ice and spun at 1,500 r.p.m. for 10 min. Nuclei were resuspended in 0.4 N H 2 SO 4 and rocked overnight at 4 °C. Histones were subsequently precipitated in 20% TCA (final concentration), spun at maximum speed for 10 min and washed sequentially with acidified-acetone and acetone. Mnase digestion and immunoblots Micrococcal nuclease treatment was performed as described [42] . Immunoblots were performed with the following antibodies: H3 C terminus (Millipore, 05–928 1:1,000), H3K4me3 (Millipore, 05–745 1:1,000), H3K9me3 (Millipore, 07–442 1:1,000), H3K14ac (Millipore, 07–353 1:5,000), H3K18ac (Millipore, 07–354 1:5,000), H3K27me3 (Millipore, 07–449 1:1,000), H3K36me2 (Millipore, 07–369 1:1,000), H3.3 (Millipore, 09–838 1:500), H4K20me3 (Millipore, 07–463 1:1,000), H3cs1 (kind gift of Dr David C. Allis 1:1,000), macroH2A1 (Millipore, 07–219 1:1,000), macroH2A2 (Bernstein Lab 1:1,000), H2A.Z (Millipore, 07–594 1:1,000), H2A.X S139ph (Cell Signaling, 97185 1:1,000), β-Actin (Sigma, A5441 1:5,000), CTSL1 (R&D systems, AF952 1:1,000), Flag (Sigma, F7425 1:1,000), MEK2 (BD BioScience, 610235 1:1,000), H-RAS (Santa Cruz Biotechnology, sc-29 1:1,000), p16 (Santa Cruz Biotechnology, sc-468 1:500), p21 (BD BioScience, 556431 1:1,000), p53 (Santa Cruz Biotechnology sc-126, 1:1,000). See Supplementary Fig. 13 for original scans of key immunoblots. Senescence assays and gene expression All senescence assays including detection of SA-β-gal, EdU incorporation, SAHF and gene expression changes were performed as described [14] . For colony formation assays, 10,000 cells per condition were plated in six-well plates and grown for 10 days post selection. Gene expression changes were measured using quantitative PCR with reverse transcription analysis. Briefly, total RNA was extracted using the RNeasy kit (Qiagen) followed by reverse transcription using SuperScript II (Life Technologies). PCRs were performed on a 7500 Fast Real Time system (Applied Biosystems) using SYBR Green Master Mix (Roche Applied Science). All values were normalized to glyceraldehyde 3-phosphate dehydrogenase and relative to the control using the ΔCT method. All quantitative PCRs were performed in triplicate. Primer sequences can be found in Supplementary Table 1 . Nevi collection Approval to collect benign nevi was granted by the Division of Dermatopathology, Icahn School of Medicine at Mount Sinai (project number 08-0964). Immunofluorescence Immunofluorescence staining was performed as described previously [40] . Briefly, cells were placed on sterilized covered slips, fixed in 4% paraformaldehyde, permeabilized with phosphate-buffered saline+0.1% or 0.5% Triton X-100 (PBST), blocked in PBST+1% bovine serum albumin or 0.5% normal goat serum and stained in the same buffer with primary and secondary antibodies before mounting onto slides. Cells were analysed using the Zeiss, Axio Imager.Z1 or Leica DMI6000B SP5 confocal system with LAS AF software. Flag antibody (Cell Signaling 2368, 1:700) and H3K9me3 (CMA318, 1:100, kind gift of Hiroshi Kimura) [43] were used for staining confocal images of SAHF. DAPI was used to visualize SAHF. RNA-seq Total RNA samples were isolated using the RNeasy kit (Qiagen) and prepared at the Icahn School of Medicine at Mount Sinai Genomics Core Facility for poly A library construction and sequencing on IlluminaHiSeq 2000. All raw RNA-sequencing reads were mapped to the human genome (hg19) with TopHat v2.0.3 (ref. 44 ) coupled with Bowtie2 (ref. 45 ) with default parameters. Transcriptomes were assembled and fragments per kilo-base per million reads for each gene were computed with Cufflinks v2.1.1 (ref. 46 ). Differentially expressed genes were identified using log2 fold change of fragments per kilo-base per million read values for all samples in pair-wise combinations. The cutoff 1.6 was used to determine lists of differentially expressed genes, as it produces lists in the hundreds range, which is suitable for enrichment and overlap analyses. ChIP enrichment analysis was carried out using the ChEA gene-set library [30] implemented within Enrichr [47] . The Fisher exact test with the Benjamini–Hochberg correction for multiple hypotheses testing was used to perform enrichment analyses. GO-enrichment analysis was carried out using DAVID [48] with default parameters. Hierarchical clustering was performed using the log2 fold change of the differentially expressed genes in senescence or the H3.3cs1 samples versus the growing control sample using MATLAB (Natick, MA). Venn diagrams were plotted to demonstrate the overlap between the identified differentially expressed genes in this study and JARID1A/1B and RB targets, as well as H3K4me3-depleted genes during senescence extracted from Chicas et al. [15] The −Log( P ) threshold for H3K4me3-depleted genes was set to 4.253 to have comparable size to the JARID1A/1B target set. Data deposition All RNA-Seq data sets have been deposited to NCBI’s Gene Expression Omnibus with the deposition number GSE55949. Native chromatin immunoprecipitation Chromatin from IMR90 cells expressing H3.1FL and H3.3cs1 was digested with MNase and used for native ChIP using H3K4me3 antibody (Abcam, ab1012), and immunoprecipitated DNA was used for qPCR essentially as described [42] . Primers were designed <1 kb downstream of the transcription start site (TSS) and controls were designed within intergenic regions. Primer sequences can be found in Supplementary Table 2 . How to cite this article : Duarte, L. F. et al. Histone H3.3 and its proteolytically processed form drive a cellular senescence programme. Nat. Commun. 5:5210 doi: 10.1038/ncomms6210 (2014).